CPEB-mediated ZO-1 mRNA localization is required for epithelial tight-junction assembly and cell polarity CPEB is a translational regulatory sequence-specific RNA-binding protein that controls germ cell development. Here we show that CPEB heterozygous female mice are fertile but contain disorganized mammary epithelial cells, in which zonal occludens-1 and claudin-3, apical tight-junction proteins, are mislocalized. CPEB depletion from mammary epithelial cells disrupts zonal occludens-1 apical localization and tight-junction distribution; conversely, ectopic expression of CPEB enhances zonal occludens-1 localization. CPEB and zonal occludens-1 mRNA are co-localized apically and zonal occludens-1 3′ untranslated region-binding sites for CPEB are necessary for RNA localization. In a three-dimensional culture system that models lumen-containing mammary ducts, depletion of CPEB or zonal occludens-1 impairs central cavity formation, indicating a loss of cell polarity. Cavity formation in zonal occludens-1-depleted cells is rescued when they are transduced with zonal occludens-1 mRNA containing, but not lacking, CPEB-binding sites. Our data demonstrate that CPEB-mediated zonal occludens-1 mRNA localization is essential for tight-junction assembly and mammary epithelial cell polarity. The asymmetric distribution of molecules in polarized cells is a hallmark of metazoan development [1] , [2] , [3] . For example, one characteristic of the anterior–posterior axis of Drosophila oocytes is the concentration of bicoid RNA at the anterior pole and oskar RNA at the posterior pole [4] . In Xenopus , oocytes are polarized along an animal-vegetal axis where RNAs [5] , [6] and organelles [7] are asymmetrically distributed. Polarization in neurons is evident not only by axonal and dendritic extensions, but also by the mRNAs that they contain [8] , [9] . Localization of molecules and subcellular structures allows cells to respond quickly and locally to environmental cues and provides a means of differentiation when cellular components are unequally distributed to cells as they divide. In mice, epithelial cells lining the lumen of several tissues are highly polarized. The mammary gland, for example, develops as a branching network of interconnecting tubular ducts that culminate in alveoli or terminal end buds (TEBs). The lumen of the ducts and TEBs become hollow when the interior most cells undergo apoptosis [10] in response to reproductive hormones [11] , [12] . The remaining epithelial cells that line the ducts become polarized with apical (luminal) and basolateral surfaces. To ensure exclusivity in the types of solutes that can passage between the lumen and the basolateral bloodstream, tight junctions are formed between cells near the apical surface [13] . Among the many factors that comprise tight junctions are the claudins, a family of 24 integral membrane proteins whose extracellular loop domains interact with one another between cells to form a selective molecular seal. The intracellular tails of the claudins contain PDZ domains (Post-synaptic density protein 95 (PSD95), Drosophila disc large tumor suppressor 1 (Dig1), and zonal occludens-1 (ZO-1)) that interact with the PDZ domains of the zonal occludens (ZO) proteins 1–3, members of the membrane-associated guanylate kinase-like homologues family of proteins. ZO-1 and ZO-2 are essential genes [14] that determine where intercellular claudin–claudin polymerization occurs and as a consequence, where tight junctions are formed. Epithelia lacking ZO-1 and ZO-2 form no tight junctions, and thus the discriminating barrier-preventing molecular mixing between luminal and basolateral regions is destroyed [14] . CPEB is a sequence-specific RNA-binding protein that regulates polyadenylation-induced translation in a variety of cell types, including germ cells [15] , [16] , neurons [17] , [18] and primary diploid fibroblasts [19] , [20] . CPEB binds the cytoplasmic polyadenylation element (CPE), a 3′ untranslated region (UTR) sequence, as well as several factors including Gld2, a poly(A) polymerase, PARN, a deadenylating enzyme, symplekin, a scaffold protein upon which the ribonucleoprotein (RNP) complex assembles, and several other factors [21] , [22] , [23] . In the nucleus, CPEB binds CPE-containing pre-mRNAs [24] , which similar to most pre-mRNAs contain long poly(A) tails, and escorts them to the cytoplasm where they associate with other members of the cytoplasmic polyadenylation complex. CPEB-bound PARN and Gld2 are constitutively active, but because PARN activity is particularly robust, the poly(A) tails are shortened. An external signal elicits CPEB phosphorylation [25] , which in turn induces the expulsion of PARN from the RNP complex resulting Gld2-catalysed polyadenylation [22] . Here we use both in vivo and in vitro models to show that CPEB controls tight-junction assembly and cell polarity by recruiting ZO-1 mRNA to the apical region of mammary epithelial cells. The involvement of CPEB in these processes establishes RNA localization by this protein as a new essential pathway for mammary cell development. Reduced TEB cavitation in CPEB-deficient mice The oocytes of CPEB knockout (KO) mice fail to progress beyond the pachytene stage of meiosis due to inefficient translation of synaptonemal complex protein mRNAs [16] , [26] , [27] . The ovaries from these sterile animals are rudimentary and do not secrete normal levels of reproductive hormones, primarily estrogen; consequently, the mammary ducts do not proliferate and elongate after birth. Although injection of 17β-estradiol for 5 days resulted in development of the mammary epithelia ( Fig. 1a ) as well as the uterus ( Supplementary Fig. S1a ), the lumen of the mammary ducts improperly contained cells ( Fig. 1a , wild type (WT) 15.2% versus KO 32.2%), suggesting that CPEB might be involved in establishing or maintaining mammary epithelial cell polarity ( Supplementary Fig. S1b,c ). There were no obvious defects in cell morphology in the kidney, intestine or liver. 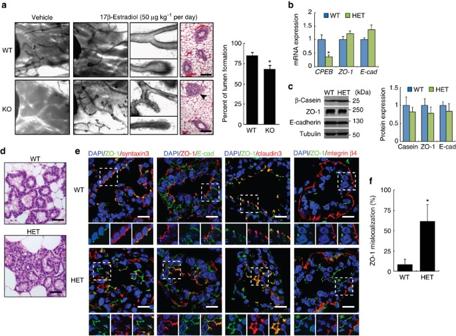Figure 1: Disruption of breast epithelial cell polarity in CPEB knockout (KO) and heterozygous mice. (a) WT and CPEB KO mice were injected with vehicle or 17β-estradiol for 5 days followed by isolation of the mammary gland, staining with Carmine's solution and examination in whole-mount, or fixation, paraffin embedding and staining with hematoxylin and eosin Y. Scale bar, 50 μm. The asterisk indicates statistical significance (P<0.05, Student'st-test, three replicates, error bars are standard error of the mean). (b,c) Quantitative reverse transcription–PCR and western blots of RNAs and proteins, respectively, in the mammary gland from WT and CPEB heterozygous (HET) mice. The asterisk indicates statistical significance (P<0.05, Student'st-test, three replicates). (d) Sections of mammary gland from WT and CPEB heterozygous mice stained with hematoxylin and eosin Y. Scale bar, 50 μm. (e) Immunostaining of WT and CPEB heterozygous mammary gland for ZO-1, syntaxin-3, claudin-3, E-cadherin (E-cad) and integrin-β4 (in this and all subsequent immunostaining, 4,6-diamidino-2-phenylindole (DAPI) co-staining indicates the nucleus). The boxes in the large merged images denote areas that are magnified and where the two fluorescent channels are separate as well as merged. Scale bar, 10 μm. (f) The percent of mislocalized ZO-1 mRNA in WT and CPEB KO mammary gland is also indicated. The asterisk indicates statistical significance (P<0.01, Student'st-test, three replicates). Figure 1: Disruption of breast epithelial cell polarity in CPEB knockout (KO) and heterozygous mice. ( a ) WT and CPEB KO mice were injected with vehicle or 17β-estradiol for 5 days followed by isolation of the mammary gland, staining with Carmine's solution and examination in whole-mount, or fixation, paraffin embedding and staining with hematoxylin and eosin Y. Scale bar, 50 μm. The asterisk indicates statistical significance ( P <0.05, Student's t -test, three replicates, error bars are standard error of the mean). ( b , c ) Quantitative reverse transcription–PCR and western blots of RNAs and proteins, respectively, in the mammary gland from WT and CPEB heterozygous (HET) mice. The asterisk indicates statistical significance ( P <0.05, Student's t -test, three replicates). ( d ) Sections of mammary gland from WT and CPEB heterozygous mice stained with hematoxylin and eosin Y. Scale bar, 50 μm. ( e ) Immunostaining of WT and CPEB heterozygous mammary gland for ZO-1, syntaxin-3, claudin-3, E-cadherin (E-cad) and integrin-β4 (in this and all subsequent immunostaining, 4,6-diamidino-2-phenylindole (DAPI) co-staining indicates the nucleus). The boxes in the large merged images denote areas that are magnified and where the two fluorescent channels are separate as well as merged. Scale bar, 10 μm. ( f ) The percent of mislocalized ZO-1 mRNA in WT and CPEB KO mammary gland is also indicated. The asterisk indicates statistical significance ( P <0.01, Student's t -test, three replicates). Full size image To investigate the possible loss of polarity further, mammary epithelia from WT and CPEB heterozygous females, which are fertile, were probed for ZO-1 and E-cadherin, two proteins involved in apical–basal epithelial cell polarity; the expression level of neither factor was altered in the heterozygote ( Fig. 1b,c ). However, the mammary epithelium from the heterozygote was often disorganized ( Fig. 1d ). Syntaxin-3 is an apical (lumenal) protein, ZO-1 and claudin-3 are essential tight-junction proteins located laterally towards the apical region, E-cadherin is an adherence junction protein located towards the basolateral region, and integrin-β4 is a basal protein. In WT mammary epithelia, these proteins segregated to their respective compartments, as expected ( Fig. 1e ). However, in the heterozygous epithelia, ZO-1 had a reduced co-localization with syntaxin-3, whereas it had an increased co-localization with E-cadherin; ZO-1 and claudin-3 remained co-localized. In WT epthelia, ZO-1 and E-cadherin immunostaining overlapped 8% of the time, whereas in heterozygous epithelia 61% of the time ( Fig. 1f ). Integrin-β4 localization was unaffected by the partial loss of CPEB ( Fig. 1e ). These data indicate that apical tight-junction assembly might be mislocalized to basolateral regions. Thus, in vivo CPEB modulates tight-junction assembly and possibly cell polarity. CPEB mediates ZO-1 localization to the apical region To examine tight-junction assembly and cell polarity in a more defined system, we used EpH4 mouse mammary cells, which were infected with lentiviruses expressing green fluorescent protein (GFP) only, or GFP plus two different short hairpin RNAs (shRNAs) targeting CPEB. Both shRNAs effectively depleted CPEB from the cells without affecting ZO-1 or E-cadherin RNA or protein levels ( Fig. 2a,b ; Supplementary Fig. S2a ). One measure of cell polarity as well as cell migration is the scratch assay, in which a wound inflicted on confluent cells is examined for repopulation. Although the rate of cell migration was unaffected by CPEB depletion, the polarity of the cells was significantly altered. As the peripheral cells migrated towards the wound, the Golgi apparatus became positioned on the leading side of the nucleus. 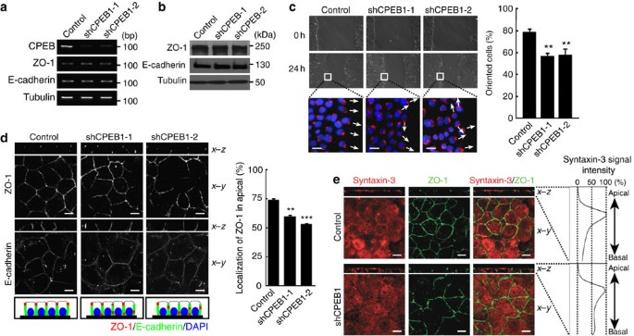Figure 2: CPEB regulates tight junctions and cell polarity of mammary epithelial cells. (a,b) EpH4 cells were infected with lentiviruses expressing GFP only or GFP plus two different shRNAs against CPEB. Reverse transcription–PCR indicates the level of CPEB RNA depletion and the western blots show the levels of ZO-1, E-cadherin or tubulin after CPEB depletion. (c) Scratch assay following CPEB knockdown. EpH4 cells infected with control or two different CPEB knockdown viruses were plated and a scratch assay performed to measure cell migration. Differential interference contrast imagines of cells 0 and 24 h after the scratch and immunostaining for GM130, a Golgi marker indicating cell polarity, are shown. The arrows indicate Golgi orientation. The histogram shows the quantification of cells that were oriented to the scratch. The two asterisks indicate statistical significance from control (P<0.01, Student'st-test, three replicates). (d) Confluent EpH4 cells infected with control or CPEB knockdown viruses were immunostained for ZO-1 and E-cadherin. The edge-on perspective of thex–zaxis shows the location of ZO-1 in apical, lateral and basal regions. Scale bar, 10 μm. The diagram illustrates the effect of CPEB depletion on ZO-1 localization and the histogram shows the quantification of ZO-1 in the apical portion of cells in thex–zaxis. The asterisks indicate statistical significance (**P<0.01; ***P<0.001, Student'st-test, three replicates). (e) Confluent EpH4 cells infected with control or CPEB knockdown viruses were immunostained for ZO-1 and syntaxin-3. The graphs representing fluorescence intensity of synatxin-3 in the apical to basal direction. Scale bar, 10 μm. Error bars are standard error of the mean. DAPI, 4,6-diamidino-2-phenylindole. Figure 2c demonstrates that in CPEB-depleted cells, the orientation of the Golgi towards the wound, as detected by GM130 immunostaining, was significantly reduced. Figure 2: CPEB regulates tight junctions and cell polarity of mammary epithelial cells. ( a,b ) EpH4 cells were infected with lentiviruses expressing GFP only or GFP plus two different shRNAs against CPEB. Reverse transcription–PCR indicates the level of CPEB RNA depletion and the western blots show the levels of ZO-1, E-cadherin or tubulin after CPEB depletion. ( c ) Scratch assay following CPEB knockdown. EpH4 cells infected with control or two different CPEB knockdown viruses were plated and a scratch assay performed to measure cell migration. Differential interference contrast imagines of cells 0 and 24 h after the scratch and immunostaining for GM130, a Golgi marker indicating cell polarity, are shown. The arrows indicate Golgi orientation. The histogram shows the quantification of cells that were oriented to the scratch. The two asterisks indicate statistical significance from control ( P <0.01, Student's t -test, three replicates). ( d ) Confluent EpH4 cells infected with control or CPEB knockdown viruses were immunostained for ZO-1 and E-cadherin. The edge-on perspective of the x – z axis shows the location of ZO-1 in apical, lateral and basal regions. Scale bar, 10 μm. The diagram illustrates the effect of CPEB depletion on ZO-1 localization and the histogram shows the quantification of ZO-1 in the apical portion of cells in the x – z axis. The asterisks indicate statistical significance (** P <0.01; *** P <0.001, Student's t -test, three replicates). ( e ) Confluent EpH4 cells infected with control or CPEB knockdown viruses were immunostained for ZO-1 and syntaxin-3. The graphs representing fluorescence intensity of synatxin-3 in the apical to basal direction. Scale bar, 10 μm. Error bars are standard error of the mean. DAPI, 4,6-diamidino-2-phenylindole. Full size image When grown in monoloayer, EpH4 cells form epithelial sheets with clearly defined tight junctions as imaged by ZO-1 immunostaining. When the images were examined along the x – z axis, ZO-1 staining was detected exclusively on the apical layer. Conversely, E-cadherin staining was mostly basolateral ( Fig. 2d ). Depletion of CPEB resulted in mislocalization of ZO-1 and claudin-3 to mid-lateral and basolateral regions; E-cadherin localization was unaffected ( Fig. 2d and Supplementary Fig. S3 , seen most clearly from the edge-on perspective of the x – z axis). A diagram of the micrographic images and quantification of the results of ZO-1 localization in the apical region are shown in Figure 2d . This ZO-1 mislocalization was not due to retardation of tight-junction assembly ( Supplementary Fig. S2b ). Another indicator of tight-junction assembly is cell permeability. In one assay, FITC-dextran applied apically to cells is measured in the medium bathing the basal surface. Relative to control, CPEB depletion resulted in greater than twofold increase in cell permeability, indicating disruption of tight junctions ( Supplementary Fig. S2c ). Taken together, these results indicate that CPEB is involved in tight-junction assembly. To examine the involvement of CPEB in cell polarity, EpH4 cells were immunostained for syntaxin-3. Figure 2e demonstrates that in control cells, syntaxin-3 was confined to the apical surface (when viewed along the x – z axis). In CPEB-depleted cells, however, syntaxin-3 was detected in apical and basal regions. Thus, CPEB mediates not only tight-junction assembly, but also cell polarity. Ectopic CPEB rescues tight junctions To determine whether CPEB might rescue tight-junction formation, EpH4 cells that were depleted of CPEB by lentivirus-mediated knockdown were subsequently infected with a retrovirus-expressing FLAG-tagged epitope (N-DYKDDDDK-C) CPEB. 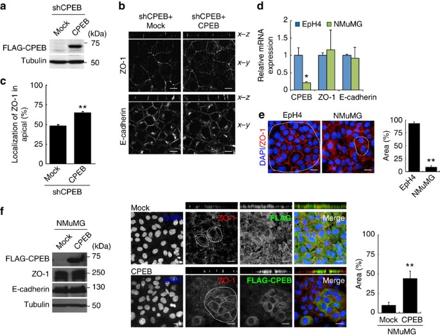Figure 3: CPEB induces ZO-1 localization to the apical surface. (a) CPEB-depleted EpH4 cells were infected with retrovirus-expressing FLAG-tagged CPEB and examined for CPEB expression by western blotting for the FLAG epitope. (b) Immunocytochemistry of ZO-1 and E-cadherin in EpH4 cells in thex–yandx–zorientations following CPEB depletion, and in some cases, following ectopic CPEB expression as well. Scale bar, 10 μm. (c) Quantification of apical ZO-1 expression. The two asterisks refer to statistical significance (P<0.01, Student'st-test, three replicates). (d) Comparison of CPEB, ZO-1 and E-cadherin expression in EpH4 and NMuMG cells by quantitative reverse transcription–PCR. The asterisk refers to statistical significance (P<0.05, Student'st-test, three replicates). (e) ZO-1 localization in EpH4 and NMuMG mammary breast epithelial cells. The circles in both cell types indicate regions that are 'EpH4-like' with ZO-1 strongly localized to apical regions. The histogram refers to the percentage of the areas that show ZO-1 apical staining. The two asterisks refer to statistical significance (P<0.01, Student'st-test, 3 replicates). Scale bar, 10 μm. (f) Expression levels of FLAG-CPEB, ZO-1, E-cadherin and tubulin in mock and FLAG-CPEB-infected cells. Also shown are NMuMG cells containing ectopically expressed FLAG-CPEB where ZO-1 protein and FLAG-CPEB were detected by immunostaining. ZO-1 localization was also examined in mock (FLAG only)-transduced cells. The circles refer to areas with strong ZO-1 localization to apical regions, and thus resemble EpH4 cells. The percent of the area of the cells that resembles the EpH4-like ZO-1 localization was quantified, which is displayed in the histogram. The two asterisks refer to statistical significance (P<0.01, Student'st-test, three replicates). Scale bar, 10 μm. Error bars are standard error of the mean. Figure 3a shows the expression of FLAG-CPEB by a western blot analysis. As presented initially in Figures 2d and 3b shows that depletion of CPEB resulted in mislocalization of ZO-1 to lateral regions (note the distribution of ZO-1 along the x – z axis). However, expression of exogenous CPEB in the depleted cells restored the apical position of ZO-1, thus demonstrating rescue of tight junctions by ectopic CPEB ( Fig. 3b,c ). Figure 3: CPEB induces ZO-1 localization to the apical surface. ( a ) CPEB-depleted EpH4 cells were infected with retrovirus-expressing FLAG-tagged CPEB and examined for CPEB expression by western blotting for the FLAG epitope. ( b ) Immunocytochemistry of ZO-1 and E-cadherin in EpH4 cells in the x – y and x – z orientations following CPEB depletion, and in some cases, following ectopic CPEB expression as well. Scale bar, 10 μm. ( c ) Quantification of apical ZO-1 expression. The two asterisks refer to statistical significance ( P <0.01, Student's t -test, three replicates). ( d ) Comparison of CPEB, ZO-1 and E-cadherin expression in EpH4 and NMuMG cells by quantitative reverse transcription–PCR. The asterisk refers to statistical significance ( P <0.05, Student's t -test, three replicates). ( e ) ZO-1 localization in EpH4 and NMuMG mammary breast epithelial cells. The circles in both cell types indicate regions that are 'EpH4-like' with ZO-1 strongly localized to apical regions. The histogram refers to the percentage of the areas that show ZO-1 apical staining. The two asterisks refer to statistical significance ( P <0.01, Student's t -test, 3 replicates). Scale bar, 10 μm. ( f ) Expression levels of FLAG-CPEB, ZO-1, E-cadherin and tubulin in mock and FLAG-CPEB-infected cells. Also shown are NMuMG cells containing ectopically expressed FLAG-CPEB where ZO-1 protein and FLAG-CPEB were detected by immunostaining. ZO-1 localization was also examined in mock (FLAG only)-transduced cells. The circles refer to areas with strong ZO-1 localization to apical regions, and thus resemble EpH4 cells. The percent of the area of the cells that resembles the EpH4-like ZO-1 localization was quantified, which is displayed in the histogram. The two asterisks refer to statistical significance ( P <0.01, Student's t -test, three replicates). Scale bar, 10 μm. Error bars are standard error of the mean. Full size image We noticed that a second murine mammary epithelial cell line, NMuMG, contained about half the amount of CPEB as EpH4 cells ( Fig. 3d ). Moreover, ZO-1 was not as tightly localized to apical tight junctions in NMuMG cells compared with EpH4 cells ( Fig. 3e ). This observation suggested that ectopic expression of CPEB in NMuMG cells might induce strong ZO-1 apical localization. Figure 3f shows the expression of FLAG-CPEB in these cells, which had little effect on the overall expression of ZO-1. However, ZO-1 in the CPEB-transduced cells was more strongly localized to the apical regions compared with neighbouring cells that did express ectopic CPEB. Moreover, in mock (FLAG only)-transduced cells, ZO-1 localization was not enhanced ( Fig. 3f ). The ZO-1 localization in the NMuMG cells that expressed ectopic CPEB resembled that of the relatively CPEB-rich EpH4 cells. Thus, ZO-1 localization, but not overall expression, is dependent upon CPEB. ZO-1 localization and cell polarity require CPEB EpH4 cells grown in an anchorage-independent manner are polarized and contain central cavities; consequently, they have been used as in vitro models to examine mammary duct formation [28] . As expected, ZO-1 was detected in the apical region ( Fig. 4a, b ). Cavity formation was strongly reduced when CPEB was depleted, but was rescued when CPEB was ectopically expressed ( Fig. 4b ). In CPEB-depleted colonies that did not form cavities, ZO-1 was randomly distributed even though steady state levels were uanffected. 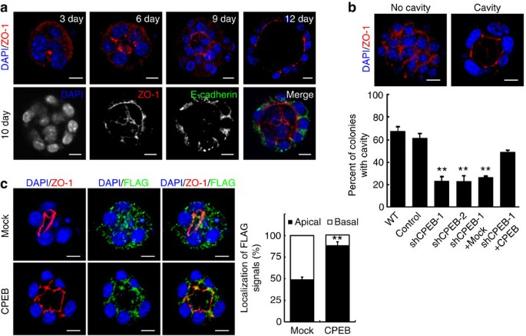Figure 4: ZO-1 localization to apical tight junctions and cavity formation require CPEB. (a) EpH4 cells were grown in suspension in Matrigel for 3–12 days. Cavity formation was monitored by immunostaining for ZO-1 and E-cadherin and examined by confocal microscopy. Scale bar, 10 μm. (b) Analysis of cavity formation in EpH4 cells cultured in Matrigel for 12 days. Scale bar, 10 μm. The histogram shows the percent of colonies with cavities following the indicated treatments. The two asterisks refer to statistical significance (P<0.01, Student'st-test, three replicates). (c) FLAG-CPEB as well as ZO-1 expression in cells that form cavities. Mock refers to cells expressing FLAG only (a nonsense protein that terminated at a stop codon in vector sequences). Scale bar, 10 μm. The histogram shows quantification of FLAG in the apical portion of cells. The asterisks refers to statistical significance (P<0.01, Student'st-test, three replicates). Error bars are standard error of the mean. DAPI, 4,6-diamidino-2-phenylindole. Figure 4: ZO-1 localization to apical tight junctions and cavity formation require CPEB. ( a ) EpH4 cells were grown in suspension in Matrigel for 3–12 days. Cavity formation was monitored by immunostaining for ZO-1 and E-cadherin and examined by confocal microscopy. Scale bar, 10 μm. ( b ) Analysis of cavity formation in EpH4 cells cultured in Matrigel for 12 days. Scale bar, 10 μm. The histogram shows the percent of colonies with cavities following the indicated treatments. The two asterisks refer to statistical significance ( P <0.01, Student's t -test, three replicates). ( c ) FLAG-CPEB as well as ZO-1 expression in cells that form cavities. Mock refers to cells expressing FLAG only (a nonsense protein that terminated at a stop codon in vector sequences). Scale bar, 10 μm. The histogram shows quantification of FLAG in the apical portion of cells. The asterisks refers to statistical significance ( P <0.01, Student's t -test, three replicates). Error bars are standard error of the mean. DAPI, 4,6-diamidino-2-phenylindole. Full size image We next infected cells with FLAG-CPEB, followed by cavity formation and immunostaining for the FLAG epitope. Compared with the FLAG epitope alone (this construct generated a nonsense protein that terminated at a stop codon in vector sequences), CPEB was at least partly co-localized with ZO-1 at the apical region of cells, significantly more that then FLAG epitope only ( Fig. 4c ). Thus, CPEB as well as ZO-1 is asymmetrically distributed to the apical region of cavity-forming cells. We also investigated whether CPEB was important for tight-junction assembly of kidney or intestinal cells grown in vitro . Madin Darby kidney cells (MDCK) and Caco-2 human colorectal epithelial cells, which contain very little CPEB RNA (only 17% and <1%, respectively, of the amount in mammary cells), were infected with lentiviruses expressing shRNA for CPEB. Supplementary Fig. S4a–d shows that these cells had normal cavity formation and ZO-1 RNA localization, indicating that CPEB involvement in these processes may be restricted to mammary cells (see Discussion ). CPEB and ZO-1 and E-cadherin mRNAs are localized apically Two observations suggest that CPEB might be involved in ZO-1 mRNA localization: CPEB is often apically co-localized with ZO-1 and ZO-1 mRNA contains five conserved CPEs in its 3′ UTR ( Supplementary Fig. S5 ). To examine this possibility, FLAG-CPEB-transduced EpH4 cells were subjected to FLAG co-immunoprecipitation and RNA analysis by reverse transcription–PCR ( Fig. 5a ). As expected, c-jun mRNA, but not tubulin mRNA, was co-immunoprecipitated with CPEB as shown previously [29] . ZO-1, ZO-2 and E-cadherin mRNAs, all of which also contain CPEs, were co-immunoprecipitated with CPEB. Other mRNAs involved in establishing cell polarity (Par-3, Par-6α, Par-6β, Par-6γ) were not co-precipitated, nor was ZO-3 mRNA. Next, cells grown without anchorage that formed a central cavity were subjected to RNA fluorescence in situ hybridization (FISH). 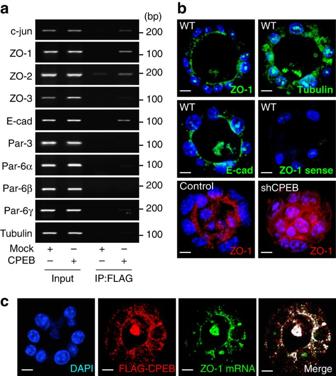Figure 5: CPEB and ZO-1 RNA co-localize at the apical region. (a) RNAs that co-immunoprecipitate with FLAG-CPEB. Input represents 10% of total RNA. Mock refers to FLAG immunoprecipitation from cells that were infected with FLAG only. (b) FISH for ZO-1, tubulin and E-cadherin mRNAs in cavity-forming cells. ZO-1 RNA was also probed with a sense strand. FISH for ZO-1 mRNA in control and CPEB knockdown cells is also shown. Scale bar, 10 μm. (c) Double staining for ZO-1 mRNA by FISH and FLAG-CPEB by immunofluorescence. Scale bar, 10 μm. Figure 5b demonstrate that ZO-1 and E-cadherin mRNAs, but not tubulin mRNA, were localized apically. A ZO-1 sense probe yielded no signal. Thus, ZO-1 mRNA is localized apically as is ZO-1 protein, but also surprisingly so too is E-cadherin mRNA even though E-cadherin protein is located basolaterally. Depletion of CPEB abolished the apical localization of ZO-1mRNA ( Fig. 5b ). Finally, a double detection of transduced FLAG-CPEB (by immunocytochemistry) and ZO-1 mRNA (by FISH) shows that these two molecules were apically localized in cavity-forming cells ( Fig. 5c ). Thus, CPEB is necessary for ZO-1 mRNA localization during as cavity formation. Figure 5: CPEB and ZO-1 RNA co-localize at the apical region. ( a ) RNAs that co-immunoprecipitate with FLAG-CPEB. Input represents 10% of total RNA. Mock refers to FLAG immunoprecipitation from cells that were infected with FLAG only. ( b ) FISH for ZO-1, tubulin and E-cadherin mRNAs in cavity-forming cells. ZO-1 RNA was also probed with a sense strand. FISH for ZO-1 mRNA in control and CPEB knockdown cells is also shown. Scale bar, 10 μm. ( c ) Double staining for ZO-1 mRNA by FISH and FLAG-CPEB by immunofluorescence. Scale bar, 10 μm. Full size image The CPE is necessary for apical RNA localization To investigate whether the CPE is involved in localizing RNA apically, GFP was fused to a portion of αCaMKII mRNA 3′ UTR, which contains two CPEs [17] and which has been shown be localized to dendrites in a CPEB-dependent manner [30] . RNA FISH performed on cavity-forming cells transduced with this construct demonstrates that the CPE mediated apical RNA localization (compare αCamKII WT with αCaMKII mutant where the CPEs were replaced by an irrelevant sequence; Fig. 6a ). In a similar experiment, GFP fused to the complete ZO-1 3′ UTR was also apically localized; in contrast, mutation of five CPEs in the ZO-1 3′ UTR significantly reduced the number of colonies with apical GFP RNA localization ( Fig. 6b ). These results demonstrate that the CPE is necessary to localize RNA to the apical portion of cells arrayed in three dimensions (3D). 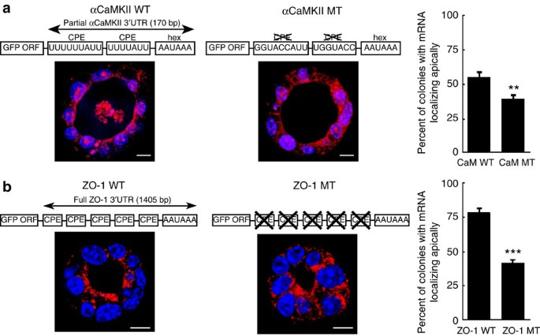Figure 6: The CPE is necessary and sufficient for RNA localization to the apical surface. (a) The GFP open reading frame was fused to a portion of the αCaMKII 3′ UTR that contains two CPEs and a polyadenylation hexanucleotide AAUAAA. For comparison, GFP was fused to an identical 3′ UTR that had the CPEs replaced with an irrelevant sequence. These constructs were transduced into cells followed by culture in Matrigel and FISH for GFP. Scale bar, 10 μm. The histogram shows the percent of colonies where the ectopic mRNA was localized apically. The two asterisks refer to statistical significance (P<0.01, Student'st-test, three replicates). (b) Cells transduced with the GFP-coding region fused to the entire ZO-1 3′ UTR, or the ZO-1 3′ UTR mutating five CPEs, were grown on Matrigel and processed for GFP FISH. Scale bar, 10 μm. The percent of colonies with GFP RNA localized to the apical surface is shown in the histogram. The three asterisks refer to statistical significance (P<0.001, Student'st-test, three replicates). Error bars are standard error of the mean. Figure 6: The CPE is necessary and sufficient for RNA localization to the apical surface. ( a ) The GFP open reading frame was fused to a portion of the αCaMKII 3′ UTR that contains two CPEs and a polyadenylation hexanucleotide AAUAAA. For comparison, GFP was fused to an identical 3′ UTR that had the CPEs replaced with an irrelevant sequence. These constructs were transduced into cells followed by culture in Matrigel and FISH for GFP. Scale bar, 10 μm. The histogram shows the percent of colonies where the ectopic mRNA was localized apically. The two asterisks refer to statistical significance ( P <0.01, Student's t -test, three replicates). ( b ) Cells transduced with the GFP-coding region fused to the entire ZO-1 3′ UTR, or the ZO-1 3′ UTR mutating five CPEs, were grown on Matrigel and processed for GFP FISH. Scale bar, 10 μm. The percent of colonies with GFP RNA localized to the apical surface is shown in the histogram. The three asterisks refer to statistical significance ( P <0.001, Student's t -test, three replicates). Error bars are standard error of the mean. Full size image CPE-dependent ZO-1 RNA localization and cavity formation We determined whether ZO-1 mRNA apical localization, which is dependent upon the 3′ UTR CPEs as well as CPEB, is necessary for cavity formation. Cells infected with a lentivirus containing an shRNA for ZO-1 were subsequently infected with a retrovirus expressing the entire ZO-1 coding sequence (1,745 amino acids) with its normal 3′ UTR (1,405 bases), or an UTR where the five CPEs were mutated. 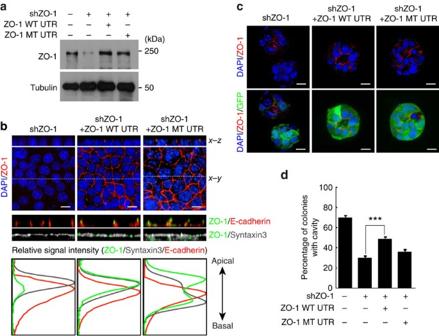Figure 7: CPE control of ZO-1 RNA localization is necessary for cell polarity. (a) EpH4 cells were infected with lentivirus expressing shRNA for ZO-1 were also transduced with retrovirus expressing the entire ZO-1-coding region plus its normal WT 3′ UTR, or an identical 3′ UTR where five CPEs were mutated (MT). The western blot shows the levels of ZO-1, with tubulin serving as a loading control. (b) Cells expressing the constructs noted inawere grown on a monolayer and then immunostained for ZO-1, E-cadherin and syntaxin-3. Confocal images are shown along thex–yandx–zaxes, where the relative fluorescence intensities of the proteins were quantified. Scale bar, 10 μm. (c) Cells expressing the same constructs as inbwere grown in an anchorage-independent manner. The cells were immunostained for ZO-1 and GFP. In the confocal images of the colonies, green indicates cells infected with shZO-1 and GFP expressing virus, red indicates immunostaining for ZO-1 and blue indicates 4,6-diamidino-2-phenylindole (DAPI). Scale bar, 10 μm. (d) The histogram shows the percent of colonies with cavities following the indicated treatments. The three asterisks refer to statistical significance (P<0.001, Student'st-test, three replicates). Error bars are standard error of the mean. Figure 7a shows ∼ 88% shRNA-mediated reduction of ZO-1, which was restored to normal levels by transduction of ZO-1 open reading frame containing its normal 3′ UTR or a UTR where the five CPEs were mutated. When grown as a monolayer and imaged along the x – z axes, ectopic ZO-1 derived from the mRNA with its WT 3′ UTR was localized to the apical surface and was indistinguishable from endogenous ZO-1 ( Fig. 7b ). In contrast, ecotopic ZO-1 derived from mRNA with the mutant 3′ UTR was detected apically and basolaterally, demonstrating that the 3′ UTR CPEs are necessary for apical localization of ZO-1. In these same cells, additional immunostaining demonstrates that ZO-1 RNA with a mutant 3′ UTR disrupted syntaxin-3 apical localization, indicating that mislocalization of ZO-1, but not depletion of ZO-1, reduces cell polarity ( Fig. 7b ). Figure 7: CPE control of ZO-1 RNA localization is necessary for cell polarity. ( a ) EpH4 cells were infected with lentivirus expressing shRNA for ZO-1 were also transduced with retrovirus expressing the entire ZO-1-coding region plus its normal WT 3′ UTR, or an identical 3′ UTR where five CPEs were mutated (MT). The western blot shows the levels of ZO-1, with tubulin serving as a loading control. ( b ) Cells expressing the constructs noted in a were grown on a monolayer and then immunostained for ZO-1, E-cadherin and syntaxin-3. Confocal images are shown along the x – y and x – z axes, where the relative fluorescence intensities of the proteins were quantified. Scale bar, 10 μm. ( c ) Cells expressing the same constructs as in b were grown in an anchorage-independent manner. The cells were immunostained for ZO-1 and GFP. In the confocal images of the colonies, green indicates cells infected with shZO-1 and GFP expressing virus, red indicates immunostaining for ZO-1 and blue indicates 4,6-diamidino-2-phenylindole (DAPI). Scale bar, 10 μm. ( d ) The histogram shows the percent of colonies with cavities following the indicated treatments. The three asterisks refer to statistical significance ( P <0.001, Student's t -test, three replicates). Error bars are standard error of the mean. Full size image When grown in an anchorage-independent manner, 70% of colonies contained cavities, which was reduced to 30% when ZO-1 was depleted. In Figure 7c , the GFP signal was a marker of the degree of ZO-1 depletion, indeed, high GFP expressing cells had reduced cavity formation. Ectopic expression of CPE-containing ZO-1 mRNA increased the colonies with cavities to 49% ( P <0.001 Student's t -test, 3 replicates), compared with shZO-1 alone, while expression of ZO-1 mRNA lacking the CPEs only modestly increased cavity formation (35%), which was statistically insignificant ( Fig. 7d ). Finally, depletion of ZO-1 had no discernible effect on E-cadherin levels, although it was not localized because of a lack of cavity formation. However, ectopic expression of ZO-1 with its WT 3′ UTR (but not its CPE-lacking 3′ UTR) in the ZO-1 shRNA-expressing cells not only restored cavity formation, but also largely restored E-cadherin localization to the basal-lateral region ( Supplementary Fig. S6 ). Thus, CPEB control of ZO-1 mRNA localization is necessary for mammary epithelial cell polarity. Because CPEB was first identified as a polyadenylation/translation factor, we used control and CPEB-depleted EpH4 cells to analyse the instantaneous synthesis of ZO-1 and E-cadherin by 35 S-methionine/ 35 S-cysteine pulse labelling followed by immunoprecipitation. In these same cells, we also examined the polyadenylation of ZO-1 mRNA and, as controls, tubulin and β-casein mRNAs. Neither the synthesis of ZO-1 or E-cadherin nor the polyadenylation of ZO-1 mRNA was affected by CEB depletion ( Supplementary Fig. S7 ) As expected, depletion of CPEB elicted reduced polyadenylation of casein mRNA [31] . Going further, we ectopically expressed CPEB with an alanine substitution for threonine 171, which renders the protein incapable of promoting polyadenylation [21] , [25] , [26] . In NMuMG cells, CPEB and CPEB T171A both promoted tight-junction assembly as evidenced by enhanced ZO-1 immunostaining ( Supplementary Fig. S8 ; Fig. 3 ). Finally, we depleted the CPEB-associated Gld2 poly(A) polymerase [21] from EpH4 cells, which also had no observable effect on tight-junction assembly or cavity formation ( Supplementary Fig. S8 ). Thus, CPEB control of mRNA localization, but not polyadenylation or translation, mediates tight-junction assembly and cell polarity. CPEB KO mice are sterile and thus do not secrete the hormones necessary for mammary duct differentiation. CPEB heterozygous mice are fertile yet their mammary ducts contain disorganized and incompletely formed TEBs. Although injection of estradiol into CPEB KO mice induces mammary formation, the lumen of the ducts and their TEBs are sometimes not fully developed. Because lumen and TEB differentiation require the establishment of tight junctions on the luminal (apical)-lateral regions of adjoining cells, we surmised that CPEB might be involved in mammary epithelial cell polarity. Indeed, CPEB is essential for polarity of mammary cells grown in monolayer (anchorage dependent) and most profoundly when grown in an anchorage-independent manner. CPEB control of polarity is mediated through ZO-1 mRNA localization; depletion of CPEB reduces apical tight-junction assembly and ZO-1 localization, although it has no effect on overall ZO-1 levels or ZO-1 RNA poly(A) tail length. The ZO-1 3′ UTR contains five CPEs that direct reporter RNAs to the apical surface. Most importantly, depletion of ZO-1 inhibits cell polarization in a 3-D culture system, which is rescued when ZO-1 mRNA containing but not lacking the CPEs is transduced into cells. These results define CPEB as a critical regulator of mammary cell polarity ( Fig. 8 ). 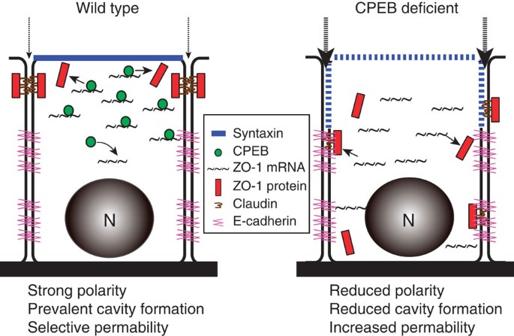Figure 8: Model depicting CPEB control of apical ZO-1 mRNA localization. The thin and thick dashed arrows refer to strong and weak tight-junction barriers to the passage of solutes in wild-type and CPEB-deficient cells respectively. Figure 8: Model depicting CPEB control of apical ZO-1 mRNA localization. The thin and thick dashed arrows refer to strong and weak tight-junction barriers to the passage of solutes in wild-type and CPEB-deficient cells respectively. Full size image Apical concentration of proteins in mammalian epithelial cells generally occurs by protein sorting rather than by mRNA localization, usually in association with the trans-Golgi network or endosomes [32] , [33] , [34] . Indeed, there is a single example, in this case in Drosophila epithelial cells of the follicle, where an alternately spliced isoform of stardust A mRNA is localized to the apical domain through an association with dynein [35] . At least in some cases, mRNA localization is thought to be determined in the nucleus, in association with exon junction complex or other proteins [36] , [37] , [38] . On protein remodelling (association or dissociation of factors) in the cytoplasm, the RNP, most likely in a translationally dormant form, coalesces with a motor protein for transport on microtubules to the ultimate destination [39] , [40] . In neurons, Xenopus oocytes, and mammalian cell lines, CPEB shuttles between nucleus and cytoplasm [24] , [41] , and likely does so in epithelial cells where it probably binds mRNA before or during export. Moreover, in neuronal dendrites, CPEB associates with kinesin and dynein is transported in both retrograde and anterograde directions [30] . We would thus anticipate that in mammary epithelial cells, CPEB also interacts with a molecular motor for apical localization. In addition to ZO-1 mRNA, CPEB binds ZO-2 mRNA, which encodes a protein that has at least a partially redundant function [14] . This observation, plus the fact that the CPE-containing PTEN is critically important for mammary epithelial cell polarity [42] suggests that CPEB control of polarity might involve these mRNAs in addition to ZO-1 (indeed, perhaps CPEB modifies the polyadenylation/translation of other such mRNAs). Moreover, it is paradoxical that CPEB binds to and co-localizes with E-cadherin mRNA in an apical domain even though E-cadherin protein resides basolaterally. We surmise that E-cadherin is synthesized apically but selectively transported to basolateral regions. In a larger sense, the presence of a CPE in an mRNA's 3′ UTR and the site of residence of the encoded protein do not necessarily go hand-in-hand. For example, the mRNA for a major apical polarity protein Par-3 has no CPE, whereas mRNAs for all three isoforms of apical Par-6 have CPEs yet none are co-immunoprecipitated by CPEB ( Fig. 5a ) and thus if they are localized, they are unlikely to be directly controlled by CPEB. Many but not all of the claudin mRNAs contain CPEs, yet probably all of these proteins are apical. Virtually, all CPE-containing mRNAs contain recognition sites for different binding proteins and miRNAs, which may displace CPEB or act singly or in combination to impart localization patterns different from ZO-1 mRNA, or indeed no localization at all. In CPEB KO mice, we detected no disruption of polarity in kidney or intestinal cells. Analysis of expression databases revealed that the level of CPEB is considerably lower in these tissues compared with mammary gland. Indeed, CPEB in MDCK (canine kidney) and Caco2 (human intestinal) epithelial cells was also low compared with EpH4 and NmuMG mammary epithelial cells. Moreover, CPEB depletion from MDCK and Caco2 cells had no discernable effect on ZO-1 localization or cell polarity. Why only mammary cell tight junctions require CPEB is not clear, but it may be related to the fact that mammary cells, but not kidney or intestinal cells, require hormonal stimulation to induce lumen formation. Perhaps CPEB responds to hormonal signalling to promote apical ZO-1 RNA localization. Indeed, cavity formation in vitro with EpH4 and NMuMG mammary cells requires hormones (insulin, corticosterone, and prolactin) in the culture medium, which is not the case with MDCK or Caco2 cells ( Supplementary Fig. S4 ). Our results generally agree with those of Umeda et al . [43] , who showed that depletion of ZO-1 did little to disrupt polarity in monolayer cells even though solute permeability was slightly increased. However, although those investigators did not examine the effect of ZO-1 deficiency in cells grown in 3D, Sourisseau et al . [44] did find that ZO-1 deficiency destroyed polarity in cells grown in Matrigel. It thus seems that 3D cell polarity is particularly sensitive to the levels and location of ZO-1 and perhaps other proteins as well. The requirement of tight junctions for establishing and maintaining cell polarity is controversial; indeed, some epithelial cells polarize even in the absence of tight junctions. On the other hand, consider the case of Par-3, a major cell polarity protein important for tight-junction assembly [45] , [46] . Ectopic expression of Par-6 disrupts the localization of Par-3 at cell–cell adhesion sites, which in turn alters tight-junction assembly as determined by mislocalization of ZO-1 (ref. 45 ). Similar experiments also show that ZO-1 mislocalization is linked to disruption of the cell polarity protein complex [47] . These data are consistent with our observations that mislocalized ZO-1 disrupts cell polarity even though deletion of ZO-1 has no effect on this process in a two-dimensional monolayer culture system. Perhaps cells lacking tight junctions compensate for cell polarity by an alternate mechanism, at least when cultured in monolayer. However, once tight junctions are mislocalized, cells lose polarity. Thus, CPEB supplies ZO-1 mRNA to apical sites to promote tight-junction assembly, and may coordinate with the Par3-aPKC pathway to establish cell polarity in mammary epithelial cells. Mouse strains and antibodies CPEB KO and heterozygous mice were generated as previously described [16] . All experiments with mice were performed according to the guidelines of the Institutional Animal Care and Use Committee of University of Massachusetts Medical School. The following antibodies were used: anti-ZO-1 (Invitrogen, for western blot 1:1,000, for immunofluorescence (IF) 1:100), anti-integrinβ4 (for IF 1:200), anti-E-cadherin (for western blot 1:2,000, for IF 1:200), and anti-GM130 (BD Transduction, for IF 1:200)), anti-claudin3 (Abcam, for IF 1:100)), anti-syntaxin3 (Synaptic system, for IF 1:100), anti-β-casein (Santa Cruz, for western blot 1:500), anti-HA (Covance, for IF 1:200), and anti-FLAG (for western blot 1:1,000, for IF 1:100) and anti-tubulin (Sigma, for western blot 1:5,000). Whole-mount mammary gland analysis Inguinal mammary glands (L4 and R4) were collected from WT and CPEB KO female mice (8 weeks) injected with 50 μg kg −1 17β-estradiol or vehicle (0.15 M. NaCl) for 5 days and from WT and CPEB heterozygous mice on day 1 of lactation. For whole-mount staining, the gland was fixed in Carnoy's solution (10% glacial acetic acid, 30% chloroform and 60% absolute ethanol), and subsequently stained in 0.2% carmine alum. For histological analysis, the gland was fixed in 4% paraformaldehyde, embedded in paraffin, sectioned and stained with hematoxylin–eosin. Mammary gland tissues were frozen using liquid nitrogen. Frozen sections were fixed in 4% paraformaldehyde, and culture cells were fixed in 3% formaldehyde for 30 min. They were permeabilized with 0.5% Triton X-100/PBS for 10 min, blocked with 2% BSA/PBS for 1 h, treated with primary antibodies for 1 h, and incubated with secondary antibodies for 1 h. They were then mounted with ProLong Gold plus DAPI (Invitrogen). Images were captured using an inverted confocal microscope. For FISH, 3D cultured cells were fixed in 3% formaldehyde for 30 min, dehydrated by successive washes in 25, 50, 75 and 100% methanol/PBST (phosphate buffered saline with Tween 20), and then rehydrated using the reverse order. Cells were acetylated in 0.25% acetic anhydride in 0.1 M triethanolamine for 10 min, treated with 10 μg ml −1 proteinase K for 10 min, stopped digestion in 2 mg ml −1 glycine/PBS for 10 min, and postfixed in 0.2% glutaraldehyde/3% formaldehyde for 20 min. Cells were prehybridized in NorthernMax hybridization buffer (Ambion), and incubated with 100 ng ml −1 fluorescein-labelled riboprobe overnight at 60 °C. After washes with 50% formamide, 1% SDS in 5× SSC (saline sodium citrate) (pH 4.5) and 50% formamide, 1% Tween-20 in 2× SSC (pH 4.5) at 60 °C, cells were blocked with 2% BSA/PBS for 1 h, and incubated with Alexa-594 conjugated anti-fluorescein antibody for 1 h. Images were captured using an inverted confocal microscope. Plasmid construction Lentiviral shRNAs targeting mouse CPEB and ZO-1 were cloned into pLentiLox 3.7. vector; shCPEB-1: 5′-GTCGTGTGACTTTCAATAA-3′, shCPEB-2: 5′-GTCCCAGAGACCCTCTAAA-3′, shZO1-1: 5′-GAGCGGGCTACCTTACTGA-3′, shZO1-2: 5′-GTGCATCTGAGATGTTTGA-3′. Human CPEB tagged with HA (YPYDVPDYA) was cloned into pOZ-C retrovirus vector, and mouse CPEB and human ZO-1 tagged with 3× FLAG were cloned into pBABE retrovirus vector. Mouse CamKII 3′ UTR with CPE (WT) or mutated CPE (MT) were cloned downstream of GFP in pBABE Mouse ZO-1 3′ UTR with CPE (WT) or mutated CPE (MT) were cloned downstream of GFP or human ZO-1 tagged with 3× FLAG in pBABE, respectively. Cell culture and virus infection Mouse mammary gland epithelial cells (EpH4 and NmuMG), dog kidney epithelial cells (MDCK) and human colorectal epithelial cells (Caco2) were maintained in DMEM containing 5 μg ml −1 insulin, 10% FBS and antibiotic-antimycotic (Invitrogen). The lentiviral and retroviral constructs were co-transfected with each packaging plasmids into 293T cells by the calcium phosphate transfection method. Virus-containing supernatants were collected 48 h after transfection, filtered to eliminate cells and target cells were infected in the presence of 6 μg ml −1 polybrene. Infected cells were selected with puromycin or sorted on a fluorescence-activated cell sorter by GFP signal intensity. For Matrigel 3D cultures, cells were trypsinized, resuspended in assay media, and plated as single cells on 100% Matrigel-coated glass cover slips in 24-well tissue culture plates. Assay media was DMEM supplemented with 2% Matrigel, 5 μg ml −1 insulin, 1 μg ml −1 hydrocortisone and 3 μg ml −1 prolactin, and changed every 3 days. To visualize changes in morphology of cavity structures, IF for ZO-1 was conducted. For calcium switching, cells were grown on glass cover slips until a monolayer was formed, and cultured in a low-calcium medium, S-MEM supplemented with 5 μM CaCl 2 and 10% FBS that had been pretreated with Chelex resin (Bio-Rad) overnight. To begin the calcium switching, the medium was replaced with normal DMEM with 10% FBS. For the wound scratch assays, EpH4 cells were grown in monolayers on glass cover slips and wounded with a pipette tip. After 24 h, cell migration and orientation was assessed. For the paracellular flux assay, cells were plated on Transwell filters 12 mm in diameter (Corning) for 6 days, and 10 μg ml −1 FITC-dextran (Sigma) was added to the medium in the apical compartment. After 1 h incubation, 100 μl aliquot of the medium was collected from the apical and basal compartment and the paracellular tracer flux was measured as the amount of FITC-dextran in the medium with a fluorometer. Immunoprecipitation of ribonucleoprotein complexes Cells were lysed in polysome lysis buffer, 10 mM HEPES-KOH pH7.0, 100 mM KCl, 5 mM MgCl 2 , 0.5% NP-40, 1 mM dithiothreitol, protease inhibitor cocktail tablets (Roche) and 100 U ml −1 RNaseOut (Invitrogen). The lysate was incubated with anti-FLAG antibody or normal IgG at 4 °C for 6 h, and further incubated with protein-G magnetic beads at 4 °C for 14 h. The beads were washed five times with polysome buffer and treated with 0.3 mg ml −1 protease K at 50 °C for 30 min. RNA was isolated using TRIZOL reagent (Invitrogen). Poly(A) and translation analysis For the poly(A) tail assay, complementary DNA was synthesized with oligo(dT) anchor primer (5′-GCGAGCTCCGCGGCCGCG-T 12 -3′), and subsequent PCR was conducted with anchor primer (5′-GCGAGCTCCGCGGCCGCG-3′) and specific primer for ZO-1 (5′-TATGGCACATCAGCACGATT-3′), tubulin (5′-CTGCTTCCACAGGGATGTTT-3′) and β-casein (5′-TTGAATTCGACCCATGGACT-3′) RNA in the presence of 32 P-ATP. For translational analysis, control and shCPEB1 infected EpH4 cells were cultured in methionine and cysteine-free media for 45 min and then cultured in media containing 100 μCi 35 S-methionine and 35 S-cysteine for 20 min. The cells were lysed in polysome lysis buffer containing protease inhibitor. The lysate was incubated with anti-ZO-1, anti-E-cadherin antibody or normal IgG at 4 °C for 6 h, and further incubated with anti-mouse IgG magnetic beads at 4 °C for 14 h. The beads were resuspended with SDS gel-loading buffer for analysis by electrophoresis and phosphorimaging. Statistical analysis Data are presented as mean±s.e.m., and Student's t -test (two-tailed) was used to compare between groups ( P <0.05 was considered significant). How to cite this article: Nagaoka, K. et al . CPEB-mediated ZO-1 mRNA localization is required for epithelial tight-junction assembly and cell polarity. Nat. Commun. 3:675 doi: 10.1038/ncomms1678 (2012).